Frequency ofTERTpromoter mutations in human cancers Reactivation of telomerase has been implicated in human tumorigenesis, but the underlying mechanisms remain poorly understood. Here we report the presence of recurrent somatic mutations in the TERT promoter in cancers of the central nervous system (43%), bladder (59%), thyroid (follicular cell-derived, 10%) and skin (melanoma, 29%). In thyroid cancers, the presence of TERT promoter mutations (when occurring together with BRAF mutations) is significantly associated with higher TERT mRNA expression, and in glioblastoma we find a trend for increased telomerase expression in cases harbouring TERT promoter mutations. Both in thyroid cancers and glioblastoma, TERT promoter mutations are significantly associated with older age of the patients. Our results show that TERT promoter mutations are relatively frequent in specific types of human cancers, where they lead to enhanced expression of telomerase. Reactivation or re-expression of telomerase is referred to be a widespread feature in human cancers, although the genetic basis remains poorly understood in many cancer types. Somatic mutations in the coding region of TERT (human telomerase reverse transcriptase) are infrequent in human tumours, but germline and somatic mutations in TERT promoter were recently found in a high percentage of human melanomas and human cancer cell lines [1] , [2] . Such mutations occurred in two hotspot positions, located −124 and −146 bp upstream from the ATG start site (−124 G>A and −146 G>A, C>T on opposite strand) and conferred enhanced TERT promoter activity [1] , [2] , by putatively generating a consensus binding site (GGAA) for ETS transcription factors within the TERT promoter region [1] , [2] . Our aim was to investigate whether the aforementioned TERT promoter mutations were present in cancer types other than melanoma, having for that matter screened 741 primary tumours from the thyroid, kidney, bladder, gastrointestinal stromal tumour (GIST), adrenal medulla (phaeochromocytomas) and central nervous system (CNS). Besides skin melanoma, we have also included ocular melanoma (not studied in the previous reports), benign lesions of the thyroid and skin and 58 human cancer-derived cell lines. Our results highlight TERT promoter mutations as frequent events in specific types of human cancers. 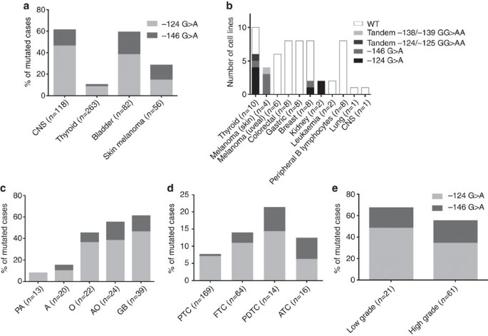Figure 1: Frequency and schematic illustration ofTERTpromoter mutations in human cancers. Graphics depict the overall frequency ofTERTmutations in the four tumour types whereTERTmutations were detected (a) and a bar plot showing the number of cell lines of different origin that harbourTERTmutations (b). The frequency and type ofTERTmutations in different histological subtypes of CNS (c), thyroid (d) and bladder (e) tumours is also shown. A, diffuse astrocytoma; AO, anaplastic oligodendroglioma; ATC, anaplastic thyroid carcinoma; GB-glioblastoma; FTC, follicular thyroid carcinoma; O, oligodendroglioma; PA, pilocytic astrocytoma; PDTC, poorly differentiated thyroid carcinoma. TERT mutations in tumours and cell lines Overall, TERT promoter mutations were found in 142 (19%) human tumour samples ( Table 1 ; Fig. 1a ) and 14 (24%) human cell lines ( Fig. 1b ; Supplementary Tables S1 and S2 ). The −124-bp mutation was the most frequent, being present in 99 cases, whereas the −146-bp mutation was present in 43 cases. The −124 G>A and −146 G>A mutations were found in a mutually exclusive fashion. Two tandem GG>AA mutations at positions −124/−125 and −138/−139 bp were observed in one cell line each ( Supplementary Fig. S1 and Supplementary Table S1 ). TERT promoter mutations were not detected in normal thyroid tissue nor in benign lesions (nevi, thyroiditis, goitres and adenomas). No mutations were detected in 26 kidney cancers, 17 phaeochromocytomas and 36 GISTs. Table 1 Prevalence of TERT promoter recurrent mutations in human cancers. Full size table Figure 1: Frequency and schematic illustration of TERT promoter mutations in human cancers. Graphics depict the overall frequency of TERT mutations in the four tumour types where TERT mutations were detected ( a ) and a bar plot showing the number of cell lines of different origin that harbour TERT mutations ( b ). The frequency and type of TERT mutations in different histological subtypes of CNS ( c ), thyroid ( d ) and bladder ( e ) tumours is also shown. A, diffuse astrocytoma; AO, anaplastic oligodendroglioma; ATC, anaplastic thyroid carcinoma; GB-glioblastoma; FTC, follicular thyroid carcinoma; O, oligodendroglioma; PA, pilocytic astrocytoma; PDTC, poorly differentiated thyroid carcinoma. Full size image TERT mutations in melanoma We have analysed both skin and ocular melanomas, a type of melanoma that was not previously studied [1] , [2] . TERT mutations were present in 16 out of 56 (29%) skin melanomas, but absent in the 25 ocular melanomas ( Table 1 ). All the four skin melanoma-derived cell lines but none of the six ocular melanoma-derived cell lines harboured TERT mutations ( Fig. 1b and Supplementary Table S1 ). Ten out of 16 (63%) skin melanomas with TERT mutation also harboured the BRAFV600E mutation, whereas the BRAF mutation was present in 9 out of 38 (24%) melanomas without TERT mutation ( P =0.01, Fisher’s exact test, two-sided) ( Supplementary Fig. S2 and Supplementary Table S3 ). TERT mutations in CNS tumours In CNS tumours, TERT promoter mutations were found in 43% (51/118) of all cases with an equal prevalence of both mutations ( Table 1 and Supplementary Table S4 ). The frequency of TERT mutations was different according to the tumour histology and grade ( Fig. 1c ): although pilocytic astrocytomas (World Health Organization (WHO) grade 1) and diffuse astrocytoma (WHO grade 2) showed a lower frequency of mutations (8% and 15%, respectively), the most aggressive form, glioblastoma multiforme (GBM; WHO grade 4), present the highest frequency of TERT mutations (62%). Oligodendrogliomas (WHO grade 2) and anaplastic oligodendrogliomas (WHO grade 3) also harboured a high frequency of TERT mutations (45% and 54%, respectively). The presence of TERT mutations was significantly associated with a higher mean age at diagnosis ( Supplementary Table S5 ) in CNS patients as a whole ( P <0.0001; Mann–Whitney test, two-tailed) and also in GBM patients only ( P =0.0247; Mann–Whitney test, two-tailed); in oligodendroglioma patients, we found the same trend, although not statistically significant ( P =0.0709; Mann–Whitney test, two-tailed). In addition, we observed that, in a subset of 14 GBM (8 TERT wild-type tumours and 6 TERT -mutated tumours), the tumours with TERT mutations showed a trend to increased immunohistochemistry (IHC) expression of telomerase, although this difference was not statistically significant ( P =0.4250; Mann–Whitney test, two-tailed) ( Fig. 2 ). 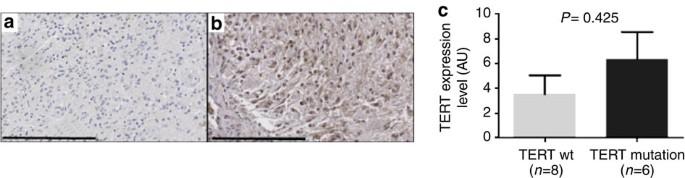Figure 2: IHC for TERT in two glioblastomas. (a)A tumour without TERT expression and withoutTERTmutation. (b) A tumour with positive staining both in nucleus and cytoplasm that also harboured aTERTmutation. The graph (c) displays quantification of TERT nuclear expression level (IHC) in glioblastomas with and withoutTERTmutation. We have measured the extent (<25%, 25–50%, 50–75% and >75%) and the intensity (absent, faint, moderate or strong) of TERT nuclear staining in 14 glioblastomas (eightTERTwild type and sixTERTmutant). The scoring was performed by two independent observers and is the product of extent and intensity of the staining (Methods). Scale bar, 200 μm. There is a trend to higher TERT expression inTERT-mutated gliomas, although the difference was not statistically significant (P=0.4250; Mann–Whitney test, two-tailed). Bars represent s.e.m. Figure 2: IHC for TERT in two glioblastomas. ( a )A tumour without TERT expression and without TERT mutation. ( b ) A tumour with positive staining both in nucleus and cytoplasm that also harboured a TERT mutation. The graph ( c ) displays quantification of TERT nuclear expression level (IHC) in glioblastomas with and without TERT mutation. We have measured the extent (<25%, 25–50%, 50–75% and >75%) and the intensity (absent, faint, moderate or strong) of TERT nuclear staining in 14 glioblastomas (eight TERT wild type and six TERT mutant). The scoring was performed by two independent observers and is the product of extent and intensity of the staining (Methods). Scale bar, 200 μm. There is a trend to higher TERT expression in TERT -mutated gliomas, although the difference was not statistically significant ( P =0.4250; Mann–Whitney test, two-tailed). Bars represent s.e.m. Full size image TERT mutations in thyroid cancer We analysed a large series of follicular cell-derived thyroid samples including normal thyroid ( n =27), benign ( n =81) and malignant lesions ( n =263) ( Table 1 and Supplementary Table S6 ). TERT mutations were only detected in malignant tumours (10%) ( Fig. 1d ), namely in 11% of papillary thyroid carcinomas (PTCs), 14% of follicular thyroid carcinomas, 21% of poorly differentiated thyroid carcinomas and 13% of the anaplastic thyroid carcinomas. Within the group of PTC, TERT mutations were detected to be associated to the so-called conventional PTC (cPTC) (11%).The majority of TERT -mutated thyroid cancers harboured the −124 G>A mutation (22 out of 27 cases) ( Fig. 1d and Supplementary Table S7 ). In thyroid cancer patients, TERT mutations were significantly associated with guarded prognosis features such as larger tumours ( P =0.008; Mann–Whitney test, two-tailed), older patients ( P <0.0001; Mann–Whitney test, two-tailed) and male gender ( P =0.0312; Fisher’s exact test, two-sided) ( Supplementary Table S5 ). After histotype stratification, such correlations were only kept in the group of cPTC where we also found significant associations with lymph node metastasis ( P =0.0318; Fisher’s exact test, two-sided) and BRAFV600E mutation ( P =0.001; Fisher’s exact test, two-sided) ( Supplementary Fig. S2 and Supplementary Table S8 ). Accordingly, we verified by quantitative RT-PCR (qPCR) that TERT mRNA is expressed at variable amounts in thyroid tumours, and the ones with coexistent TERT and BRAF mutations showed the highest levels of TERT mRNA expression ( P =0.0001, unpaired t -test; Fig. 3 ). 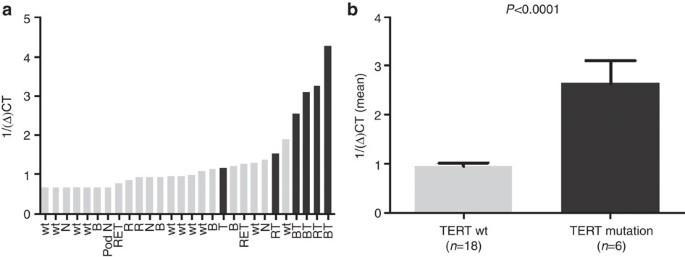Figure 3: Quantification ofTERTmRNA expression level in thyroid tumours. We have performed qPCR in normal thyroid tissue (N), a pool of mRNA of nine normal thyroids (pool N) and thyroid tumours with different genetic backgrounds: without known genetic alterations (wt), withBRAFmutation (B), withRETrearrangement (RET), withRASmutation (R), withTERTmutation (T), withTERTandBRAFmutations (BT) or withRASandTERTmutations (RT). (a) Each bar representsTERTmRNA expression in an individual tumour measured in triplicate.TERTmRNA levels were normalized againstTBPmRNA levels. (b) Quantification ofTERTmRNA mean expression level in thyroid tumours with and withoutTERTmutation. Error bars represent s.e.m. The difference is statistically significant (P<0.0001, unpairedt-test). Figure 3: Quantification of TERT mRNA expression level in thyroid tumours. We have performed qPCR in normal thyroid tissue (N), a pool of mRNA of nine normal thyroids (pool N) and thyroid tumours with different genetic backgrounds: without known genetic alterations (wt), with BRAF mutation (B), with RET rearrangement (RET), with RAS mutation (R), with TERT mutation (T), with TERT and BRAF mutations (BT) or with RAS and TERT mutations (RT). ( a ) Each bar represents TERT mRNA expression in an individual tumour measured in triplicate. TERT mRNA levels were normalized against TBP mRNA levels. ( b ) Quantification of TERT mRNA mean expression level in thyroid tumours with and without TERT mutation. Error bars represent s.e.m. The difference is statistically significant ( P <0.0001, unpaired t -test). Full size image TERT mutations in bladder cancer In bladder cancer, TERT mutations were frequently detected (48/82; 59%) both in low-grade tumours (14/21; 67%) and high-grade tumours (34/61; 56%) ( Table 1 and Fig. 1e ; Supplementary Table S9 ). The −124 G>A mutation was present in 30 cases, whereas the −146 G>A was found in 18 cases. No association was found between the presence of the mutation and the age of the patients. No mutations were detected in 26 kidney cancers, 17 phaeochromocytoma and 36 GISTs ( Supplementary Tables S10, S11 and S12 , respectively). Recent findings have described that TERT promoter mutations arise as a novel mechanism of telomerase reactivation/expression in human cancers [1] , [2] . In this work, we report for the first time the presence of these mutations in different histotypes of thyroid cancer, and our results validate the findings reported by others in melanoma, bladder and gliomas [1] , [2] , [3] . Furthermore, we present for the first time evidence showing that TERT promoter mutations are significantly associated with increased TERT mRNA expression in thyroid cancers. We also found a trend for increased telomerase expression in cases of GBM harbouring TERT promoter mutations. In thyroid cancers, TERT mRNA was particularly high in cases harbouring both TERT and BRAF mutations. The location of these mutations in the TERT promoter, rather than the coding region of the gene, creating additional binding sites for transcription factors, represents also a novel mechanism of genetic activation in cancer. The frequency of TERT mutations we detected in skin melanomas is similar to that reported by Horn et al . [1] in primary melanomas (33%), but lower than the frequency found by the same authors in metastatic melanomas (85%) and by Huang et al . [2] in a series of 70 melanomas and short-term cultures [1] , [2] . In our series, we have analysed few metastatic melanomas that did not show a significantly higher percentage of TERT mutations. As our series is too small to allow a conclusion, it remains to be verified if there is an increased frequency of TERT mutations in metastatic melanomas, as suggested by previous reports [1] , [2] . We have confirmed, in skin melanomas, the significant association between TERT and BRAF mutations, as previously advanced by Horn et al . [1] , which we now also demonstrate in thyroid cancers. Interestingly, in benign nevi, which frequently harbour BRAF mutations, we did not detect TERT mutations. This finding, together with the high frequency of TERT mutations in metastatic melanomas [1] , suggests that, although BRAF mutations are thought to be an early event in melanoma genesis, TERT mutations may occur at a later stage. No TERT promoter mutations were found in ocular melanomas, which, at variance with skin melanomas, harbour GNAQ mutations instead of BRAF mutations [4] , [5] . Our results further support the assumption that ocular melanomas result from different etiopathogenic mechanism than skin melanomas [5] , [6] . Our data on CNS tumours indicate that TERT promoter mutations are frequent events in gliomas, particularly in GBM where the highest mutation frequency was found. It has been shown that TERT mutations conferred enhanced TERT promoter activity in vitro [1] , [2] ; our findings fit with this assumption because we observed that GBM with TERT promoter mutations appear to display increased telomerase expression, despite the limited sensitivity of IHC and the low number of cases analysed. Our results are also in concordance with those of Lotsch et al . [7] who reported that 60% of GBMs were positive for TERT mRNA and telomerase activity [7] . It will be interesting to assess whether the GBM positive for telomerase activity described by Lotsch et al . [7] also harbour TERT promoter mutations. Our findings also indicate that TERT mutations are associated with older patients, in accordance with a recent report [3] . The high frequency of TERT mutations in CNS tumours, particularly in intermediate and high-grade tumours, opens a window for new approaches in the therapy of CNS tumours. In thyroid cancer, TERT mutations were only found in follicular cell-derived cancers (PTC, follicular thyroid carcinoma, poorly differentiated thyroid carcinoma and anaplastic thyroid carcinoma). No mutations were detected in medullary thyroid carcinomas, as described by Killela et al . [3] , nor in normal thyroid and benign lesions, such as goitre, adenomas or thyroiditis; this finding fits with previous studies that reported telomerase expression in malignant lesions and not in normal tissue or hyperplastic lesions [8] , [9] . TERT mutations were associated with clinicopathological features (older age, increased tumour size and male gender), but, after histotype stratification, these associations were only maintained in cPTC. Studies in larger series will be necessary to clarify these associations. In cPTC, TERT mutations were associated with BRAF mutation, highlighting the coexistence of activation of BRAF and TERT , previously reported in melanoma [1] ( Supplementary Fig. S2 ). Our results reinforce the hypothesis of a link between BRAF activation and telomerase expression, which can be mediated by transcription factors binding to the newly created consensus binding sites, as previously advanced by Horn et al . [1] . Both in thyroid carcinoma and melanoma, it seems that a ‘background’ status of activated BRAF enhances the effects of TERT promoter mutation. Our results in TERT mRNA expression strengthen this assumption, showing, for the first time, an increased TERT expression in tumours harbouring BRAF and TERT mutation ( Fig. 3 ). Further observational and mechanistic studies are needed to clarify these points. TERT alterations seem to constitute an early and frequent event in bladder cancer. These findings fit with the high prevalence of telomerase activity previously described in bladder tumours [10] . The recurrent hotspot mutations in TERT were advanced to be, in melanomas, induced by ultraviolet radiation [2] . Bladder is a target for several chemical carcinogens; it remains to be found whether TERT mutations can also result from the action of such agents. The identification of TERT mutations in urine may provide a biomarker for early diagnosis and monitoring of bladder cancer. No TERT mutations were detected in kidney cancers, nor in 17 phaeochromocytoma and 36 GISTs. The underlying reasons for the tissue specificity of TERT mutations remain to be clarified. We can hypothesize that TERT mutations can be present in two settings. As described by Killela et al . [3] , TERT mutations can be relevant in tissues with relative low rates of self-renewal, which fits with our findings in follicular cell-derived thyroid cancer and gliomas where they are associated with the older age of the patients. On the other hand, these mutations can also result from environmental factors such as ultraviolet radiation and chemical carcinogens as suggested by their high frequency in melanoma, bladder and tongue [1] , [2] , [3] . In summary, our data identify TERT mutations as common events in human cancers and support the assumption that TERT promoter mutations may be one of the mechanisms that underlies telomerase reactivation in several types of human tumours. Human cancer samples All the procedures described in this study were in accordance with national and institutional ethical standards and previously approved by Local Ethical Review Committees. According to Portuguese law, informed consent is not required for retrospective studies. Formalin-fixed, paraffin-embedded tissues from nine cases of sporadic nevi, 56 cases of sporadic skin melanomas and 25 cases of ocular melanoma were retrieved from the files of the Hospital S. João (HSJ)/Medical Faculty of Porto (FMUP), Porto, Portugal, the Department of Pathology of HSJ and the Department of Pathology of Hospital S. Marcos (HSM), Braga, Portugal. Clinicopathological and follow-up data were retrieved from the files of the Department of Pathology, Department of Dermatology and Oncology Registry of HSJ and Department of Pathology of HSM, and from RORENO (Oncology Registry of North Region). All skin melanoma cases were re-evaluated and staged according to the seventh edition of the American Joint Committee on Cancer [11] . The overall female:male ratio was 1.2:1. The mean age of the patients was 58 years for females (s.d.±17.6), with a range from 9 to 94 years, and 62 years for males (s.d.±13.1), with a range from 33 to 79 years. Follow-up data were available for 53 patients, including the diagnosis of metastases, through the evaluation of the patients or direct interview with their relatives and by review of in-hospital patient files/RORENO. The mean follow-up time of patients was 41 months (range 1–170). During follow-up, 5 (9%) patients developed (lymph node, liver or brain) metastases and 8 (15%) patients died due to malignant melanoma. The remaining patients were alive and without evidence of melanoma recurrence at the last follow-up. Additional information regarding the melanoma subtype, age, gender, thickness and molecular analysis of TERT , BRAF and NRAS is compiled in Supplementary Table S3 . Formalin-fixed, paraffin-embedded tissues from 372 tumours and tumour-like lesions of the thyroid and 27 normal thyroids were collected from the files of IPATIMUP, HSJ/FMUP and the Portuguese Institute of Oncology, Coimbra, Portugal. The histology of all tumour samples was revised, and the final classification was made according to the WHO criteria [12] . In Supplementary Tables S6 and S7 , we have summarized the information regarding histological classification of the lesions, gender, mean age of the patients, molecular data and the size of the tumours. Representative formalin-fixed paraffin-embedded samples from 118 gliomas were retrieved from pathology archives of the Department of Pathology of HSJ/FMUP and the Department of Pathology of HSM, Braga, Portugal. The tumours were reviewed and classified according to the WHO classification of CNS tumours (2007) (ref. 13 , 14 ). This cohort includes lesions that were classified as pilocytic astrocytoma ( n =13), astrocytoma grade 2 ( n =20), oligodendroglioma ( n =22), anaplastic oligodendroglioma ( n =24) and glioblastoma ( n =39). Further information regarding the CNS cases is available in Supplementary Table S4 . Formalin-fixed, paraffin-embedded tissues were collected from 82 patients with non-muscle invasive bladder cancer who underwent transurethral resection of the bladder malignant tumours in the Portuguese Institute of Oncology, Porto. Haematoxylin–eosin-stained sections were reviewed according to the standard histopathological examination by two independent pathologists. Staging and grading were conducted according to the American Joint Committee on Cancer [11] , and the 2004 WHO classification system [15] . Supplementary Table S9 summarizes the clinicopathological parameters. Formalin-fixed, paraffin-embedded tissues from 26 kidney cancers were collected from the HSJ/FMUP. Cases were classified as clear cell renal cell carcinoma ( n =12), chromophobe renal cell carcinoma ( n =4) and papillary renal cell carcinoma ( n =10). Information addressing the diagnosis, age, gender, nuclear grade and staging is obtainable in Supplementary Table S10 . Formalin-fixed, paraffin-embedded tissues from 17 pheochromocytomas were collected from the HSJ/FMUP and IPATIMUP, Porto, Portugal. Supplementary Table S11 summarizes the clinicopathological parameters. Formalin-fixed, paraffin-embedded tissues from 36 GIST were collected from the HSJ/FMUP and IPATIMUP, Porto, Portugal. Tumours were classified according to the WHO pathological classification [16] , and the parameters analysed in each case included: age, gender and tumour size. These data and the molecular characterization of these tumours can be observed in Supplementary Table S12 . Cell lines DNA from 58 cell lines deposited in IPATIMUP cell line bank was retrieved. All the cell lines were authenticated using DNA profile analysis, obtained with the PowerPlex 16 system (Promega, Madison, USA), according to the DNA profiles available in American Type Culture Collection and Health Science Research Resource Bank. DNA extraction DNA from formalin-fixed, paraffin-embedded tissues was retrieved from 10-μm cuts after careful microdissection. DNA extraction was performed using the Ultraprep Tissue DNA Kit (AHN Biotechnologie, Nordhausen, Germany) following the manufacturer’s instructions. RNA extraction Total RNA was extracted from frozen thyroid tumours ( n =24) and normal tissue specimens ( n =3) using a Trizol commercial kit (Life Technologies, GIBCO BRL, Carlsbad, CA) according to the manufacturer’s protocol. RNA was quantified spectrophotometrically, and its quality was checked by analysis of 260/280ηm and 260/230 ηm ratios. PCR and Sanger sequencing Coding regions of BRAF, GNAQ HRAS, NRAS, cKIT and PDGFR were screened for mutations in DNA extracted from paraffin blocks using PCR and Sanger sequencing. The genetic characterization of part of the tumours had already been previously reported. For information on primers and PCR conditions, see refs 5 , 17 , 18 . To screen for TERT promoter mutations, we analysed the hotspots previously identified by PCR followed by Sanger sequencing. TERT promoter mutation analysis was performed with the pair of primers FwTERT: 5′-CAGCGCTGCCTGAAACTC-3′ and RwTERT: 5′-GTCCTGCCCCTTCACCTT-3′. Amplification of genomic DNA (25–100 ng) was performed by PCR using the Qiagen Multiplex PCR kit (Qiagen, Hilden, Germany) according to the manufacturer’s instructions. Sequencing reaction was performed with the ABI Prism BigDye Terminator Kit (Perkin-Elmer, Foster City, CA), and the fragments were run in an ABI prism 3100 Genetic Analyser (Perkin-Elmer). The sequencing reaction was performed in a forward direction, and an independent PCR amplification/sequencing, both in a forward and reverse direction, was performed in positive samples or samples that were inconclusive. Quantitative RT-PCR qPCR for human TERT was performed in 28 thyroid samples, 24 tumours and 3 normal tissue specimens. We also included a normal reference that was produced by pooling RNAs from nine samples of normal thyroid tissue [19] . For cDNA preparation, 1 μg of total RNA was reverse transcribed using the RevertAid first strand cDNA synthesis kit (Fermentas, Burlington, ON, Canada). Reverse transcription products were amplified for the TERT by qPCR (IDT; no. HS.PT.56a.40988589) using TaqMan PCR Master Mix (Applied Biosystems, Foster City, CA, USA) with TBP gene (TATA-binding protein) as endogenous control (Applied Biosystems; no. 4326322E-0705006). The ABI PRISM 7500 Fast Sequence Detection System (Applied Biosystems) was used to detect the amplification level and was programmed to an initial step of 2 min at 50 °C, 10 min at 95 °C, followed by 45 cycles of 95 °C for 15 s and 60 °C for 1 min. TBP and TERT amplifications were done in triplicate using 1 μl of cDNA (~50 ng) for each sample. The relative quantification of target genes was determined using the ΔΔCT method, which was previously validated by Livak’s Linear Regression Method (slope=0.0696) (Sequence Detector User Bulletin 2; Applied Biosystems). Immunohistochemistry IHC for telomerase was performed in representative tumour tissue sections of 14 glioblastomas. Briefly, deparaffinized and rehydrated sections were subjected to microwave treatment in 10 mM sodium citrate buffer, pH 6.0, for antigen retrieval. The sections were incubated overnight at 4 °C in a humidified chamber with the primary antibody telomerase (polyclonal, rabbit, 1:500) from Rockland Immunochemicals Inc., Gilbertsville, PA. The detection was performed with a labelled streptavidin–biotin immunoperoxidase detection system (Thermo Scientific/Lab Vision, Fremont, USA), and the immunohistochemical staining was developed with 3,3′-diaminobenzidine substrate. Omission of the primary antibody incubation was used as negative control. Previously tested liver cancer case was used as positive control. IHC evaluation was performed independently by two observers (V.M. and J.L.). An IHC score was established, which corresponded to the product of the intensity of expression (absent=0, faint=1, moderate=2 and strong=3) with the tumour extent of protein expression (0–25%=0, 26–50%=1, 51–75%=2 and >75%=3) (ref. 6 ). Statistical analysis Statistical analysis was conducted with StatView for Windows, version 5.0 (SAS Institute, Cary, NC). The results are expressed as a percentage or mean±s.d. Statistical analysis was performed both on the whole series and considering the different groups of lesions. For the analysis of the relationship between patients’ age, tumour size and TERT status of the tumours, we used the unpaired t -test, Mann–Whitney test and analysis of variance. Fisher’s exact test was used in the statistical analysis of the other parameters. Graphs and figures were done in GraphPad v6.0. Results were considered statistically significant if P <0.05. How to cite this article: Vinagre, J. et al . Frequency of TERT promoter mutations in human cancers. Nat. Commun. 4:2185 doi: 10.1038/ncomms3185 (2013).